Unveiling pseudospin and angular momentum in photonic graphene Pseudospin, an additional degree of freedom inherent in graphene, plays a key role in understanding many fundamental phenomena such as the anomalous quantum Hall effect, electron chirality and Klein paradox. Unlike the electron spin, the pseudospin was traditionally considered as an unmeasurable quantity, immune to Stern-Gerlach-type experiments. Recently, however, it has been suggested that graphene pseudospin is a real angular momentum that might manifest itself as an observable quantity, but so far direct tests of such a momentum remained unfruitful. Here, by selective excitation of two sublattices of an artificial photonic graphene, we demonstrate pseudospin-mediated vortex generation and topological charge flipping in otherwise uniform optical beams with Bloch momentum traversing through the Dirac points. Corroborated by numerical solutions of the linear massless Dirac-Weyl equation, we show that pseudospin can turn into orbital angular momentum completely, thus upholding the belief that pseudospin is not merely for theoretical elegance but rather physically measurable. Graphene, a two-dimensional honeycomb lattice of carbon atoms, has been highly touted and tested as an extraordinary material for many applications, apart from elucidating fundamental phenomena in quantum and condensed matter physics [1] , [2] , [3] , [4] . Central to this enthusiasm is the unique electronic band structure of the graphene lattice, which exhibits a linear energy dispersion relation in the vicinity of the so-called Dirac points. Electrons around these Dirac points behave as massless relativistic particles. Although extracting a single atomic layer of graphite (as ‘natural’ carbon-based graphene) can be readily accomplished nowadays with simple laboratory techniques [3] , there is a surge of interest recently in creating ‘artificial’ graphene systems; not only for electrons but also for atoms, photons and polaritons. These include, for example, nanopatterning of two-dimensional electron gases, assembling molecules on metal surfaces, trapping ultracold atoms in optical lattices and engineering coupled micropillars in semiconductor microcavities [5] , [6] , [7] , [8] , [9] , [10] , [11] , [12] , [13] . Artificial graphene can provide a tunable platform to explore physical phenomena that are otherwise difficult or impossible to achieve in natural graphene. In particular, photonic graphene (a honeycomb array of evanescently coupled waveguides [14] ) has proven to be a useful tool for investigating graphene physics in various optical settings [15] , [16] , [17] , [18] , [19] , [20] , [21] , [22] , [23] . As photonic lattices offer exquisite control over initial conditions and allow for monitoring the actual wavefunction (including phase), it is possible to directly observe graphene wave dynamics using classical light waves in regimes not accessible in natural graphene. Exemplary successes include the recent demonstrations of defect-free Tamm-like edge states [20] , [21] , strain-induced pseudomagnetic fields and photonic Landau levels [22] , and the photonic Floquet topological insulators [23] . Another intriguing concept in graphene is the ‘pseudospin’, introduced initially due to the mathematical analogy between the graphene sublattice degree of freedom and the electron spin in the original Dirac equation. It has certainly turned into one of the paradigms of graphene physics [1] , [2] , [3] , [4] . Although recent experiments with angle-resolved photoemission spectroscopy has led to direct probing of the Berry phase in graphene systems [24] , the pseudospin itself is considered to be unmeasurable. This is simply because that, unlike the electron spin, the pseudospin is not detectable by any magnetic field even if it corresponds to an angular momentum (AM) [25] , [26] . In this letter, by use of photonic graphene as a test bed, we investigate the pseudospin and its associated AM. In our optical setting, we can selectively excite each of the two sublattices of photonic graphene, breaking the degeneracy introduced by the two inequivalent atomic sites in the honeycomb lattice (HCL), and thus unveiling the underlying physics of pseudospin. Specifically, we employ two different methods to alternatively excite one of the two sublattices forming the photonic graphene, and observe the vortex generation when an initially vortex-free probe beam with Floquet momentum in the vicinity of the Dirac points travels through the lattice. Moreover, the topological charge of the generated vortex flips as the excitation of the probe beam moves from one sublatttice to another. By comparing our experimental results with numerical and theoretical analyses of the linear massless Dirac-Weyl equation, we show that the observed vortices (optical beams carrying orbital AM [27] ) are a direct consequence of the AM transfer from the lattice to the probe beam. Unlike the electron spin, such pseudospin AM is not associated with any intrinsic property of particles, but rather arises from the substructure in space (sublattices) that the particles (or wave packets) live in. Our work may lead to new insights of pseudospin-mediated fundamental phenomena in both natural and artificial graphene systems. Pseudospin-mediated vortex generation by three-beam excitation The HCL is composed of two inter-penetrating triangular sublattices, whose representing lattice sites are denoted by A and B as shown in Fig. 1a . The band gap structure β ( k x , k y ) plotted in Fig. 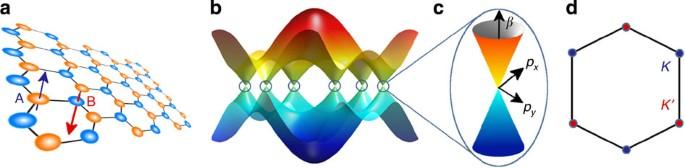Figure 1: Schematic of the lattice and band structure of the honeycomb lattice. (a) Honeycomb lattice structure of graphene, where arrows illustrate the pseudospin representation of honeycomb sublattice (A or B) degree of freedom. (b) The band gap structure of graphene lattice exhibiting six Dirac points. (c) Zoom-in of the linear dispersion close to one of the Dirac points. (d) The first Brillouin zone of the lattice where the locations of two inequivalent corners are marked byKandK′. 1b is calculated from the following paraxial Schrödinger-type equation describing light propagation in the photonic lattice [14] : Figure 1: Schematic of the lattice and band structure of the honeycomb lattice. ( a ) Honeycomb lattice structure of graphene, where arrows illustrate the pseudospin representation of honeycomb sublattice (A or B) degree of freedom. ( b ) The band gap structure of graphene lattice exhibiting six Dirac points. ( c ) Zoom-in of the linear dispersion close to one of the Dirac points. ( d ) The first Brillouin zone of the lattice where the locations of two inequivalent corners are marked by K and K ′. Full size image where Ψ is the electric field envelope of the probe beam, x, y are the transverse coordinates, z is the longitudinal propagation distance, k 0 is the wavenumber, n 0 is the background refractive index of the medium, and Δ n is the induced index change forming the HCL. In equation (1), H 0 is the continuous Hamiltonian of the system, whose eigenvalues are the wavenumbers along the z -direction (that is, the propagation constant β ). From Fig. 1b , one can see clearly the touching of two bands at the six Dirac points, where the Floquet-Bloch dispersion relation is linear ( Fig. 1c ). These Dirac points are located at the corners of the first Brillioun zone (BZ) of the HCL, noted as K and K ′ in Fig. 1d . Applying the coupled mode theory (under the tight-binding approximation) to equation (1), one can obtain a two-band simplified description of the paraxial model [17] . In the continuous limit and for excitations near the Dirac points, the coupled mode equation turns into the linear Dirac equations typically used for describing massless Dirac particles in graphene: where μ =(−1) m =±1, and m =0,…,5 is the index of the six Dirac points shown in Fig. 1d . The associated Hamiltonian can be written as H = σ y p x − μσ x p y , where p =( p x , p y ) is the Bloch momentum measured from the Dirac points, σ =( σ x , σ y ) are the Pauli matrices [3] . Detailed derivations and analysis of equation (2) are presented in the Supplementary Information section. Thus, an optical beam with Bloch momentum at the close vicinity of Dirac points is governed by the Dirac equation, akin to massless Dirac Fermions in graphene. The amplitude of the optical wave in the spatially separated sublattice sites (marked as A and B in Fig. 1a ) is modelled by the two-component spinor function with components ψ A and ψ B , respectively. Therefore, as we shall elaborate below, the sublattice states play the role of electron spins, typically referred to as ‘pseudospin’. In light of such an analogy, a natural question arises: is the lattice spin associated with real AM [25] observable in our optical setting? To answer the above question, we first perform a numerical beam propagation simulation of the paraxial equation (equation (1)) to illustrate the pseudospin-mediated vortex generation by sending three interfering plane waves as a probe to the HCL ( Fig. 2a ). The three input wave vectors point at three alternative Dirac points ( K or K ′), thus the two sublattices can be selectively excited by the probe beam, which exhibits a triangular lattice pattern ( Fig. 2e ). Specifically, in the first setting (three waves of equal phase), only sublattice A is excited ( Fig. 2b ). In the second setting (three waves of a 2π/3 phase difference in k -space), only sublattice B is excited but not sublattice A ( Fig. 2f ). Surprisingly, although the output intensity of the probe beam displays a similar conical diffraction pattern [14] , [28] as shown in Fig. 2c,g , their phase structure as monitored from interferograms is dramatically different. In both cases, a global singly charged vortex is created, as identified by a fork bifurcation in the central fringes, although the topological charges are opposite ( Fig. 2d,h ). It should be noted that the input beam initially contains no phase singularity. In addition, when both sublattices A and B are simultaneously excited or when the HCL is replaced by a single triangular lattice, no integer vortex is generated. These results suggest that the vortex generation and topological charge flipping is a direct consequence of the special symmetry and sublattice degree of freedom of the HCL, which will be confirmed later by introducing the total AM and directly solving the Dirac equation. 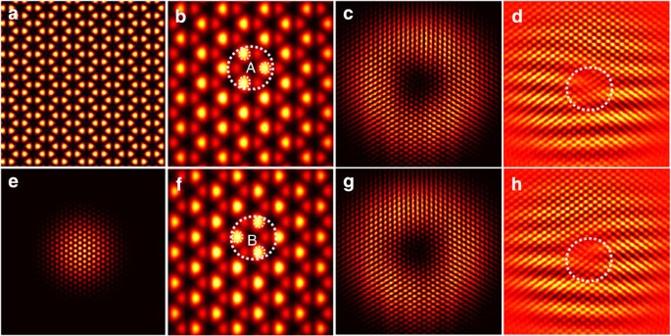Figure 2: Numerical simulation of pseudospin-mediated vortex generation in photonic graphene. (a) The honeycomb lattice, and (e) the input triangular lattice as a probe formed by three-beam interference. (b,f) Superimposed patterns (zoomed in) when only sublattice A (top row) or B (bottom row) is excited. The output intensity patterns of the probe beam exhibit similar conical diffraction (c,g), but the interferograms obtained with an inclined plane wave reveal opposite phase singularities in the centre (d,h) due to excitation of different pseudospin states (Parameters for simulation are chosen close to those from experiment: the lattice spacing is 7 μm, the strength of refractive index modulation is 2 × 10−4and the propagation distance is 20 mm). Figure 2: Numerical simulation of pseudospin-mediated vortex generation in photonic graphene. ( a ) The honeycomb lattice, and ( e ) the input triangular lattice as a probe formed by three-beam interference. ( b , f ) Superimposed patterns (zoomed in) when only sublattice A (top row) or B (bottom row) is excited. The output intensity patterns of the probe beam exhibit similar conical diffraction ( c , g ), but the interferograms obtained with an inclined plane wave reveal opposite phase singularities in the centre ( d , h ) due to excitation of different pseudospin states (Parameters for simulation are chosen close to those from experiment: the lattice spacing is 7 μm, the strength of refractive index modulation is 2 × 10 −4 and the propagation distance is 20 mm). Full size image Next, we experimentally demonstrate the pseudospin-mediated vortex generation in a photonic graphene system—the HCL is created by optical induction, which translates lattice intensity pattern into refractive index change in a photorefractive nonlinear crystal [29] , [30] , [31] , [32] . A detailed description of the experimental setup is given in the Methods section. Typical results are shown in Figs 3 and 4 , which correspond to two different methods of selectively exciting the two graphene sublattices. The index change associated with the HCL is about 1.5 × 10 −4 , and the lattice constant is about 7 μm ( Fig. 3a ). The BZ spectrum of the induced lattice shown in Fig. 3b is measured separately using BZ spectroscopy with incoherent light [33] . In the first method, three broad Gaussian beams forming a triangular lattice pattern ( Fig. 3e ) are carefully aimed onto the three Dirac points in the first BZ ( Fig. 3f ). To selectively excite the two sublattices in the same experimental setting, the probe lattice has the same period as the sublattices and it can be readily translated along the transverse direction by moving the focus lens. Note that the intensity/polarization of all beams is chosen such that there is no nonlinear self-action of the probe beam. Clearly, when the probe beam excites only sublattice A ( Fig. 3c ) or sublattice B ( Fig. 3g ), there is not much difference in the output intensity pattern after propagating 2 cm through the HCL, as in both cases the beam exhibits a low intensity in central region due to conical diffraction. However, the interferograms obtained with an inclined reference plane wave indicate that not only is a singly charged optical vortex created in each case, but also the topological charge is flipped (opposite fringe bifurcation) when the excitation shifts from sublattice A to B ( Fig. 3d,h ). Under the same excitation condition, if the HCL is reconfigured into a single triangular lattice (that is, only one sublattice is present), no fringe bifurcation is observed in the interferograms. Likewise, when the HCL is completely blocked, the three input beams propagate independently and no vortex is observed whatsoever. These simple tests indicate clearly that the observed vortex is not in any way related to experimental artefacts. In fact, our experimental observations agree well with the simulation results of Fig. 2 . 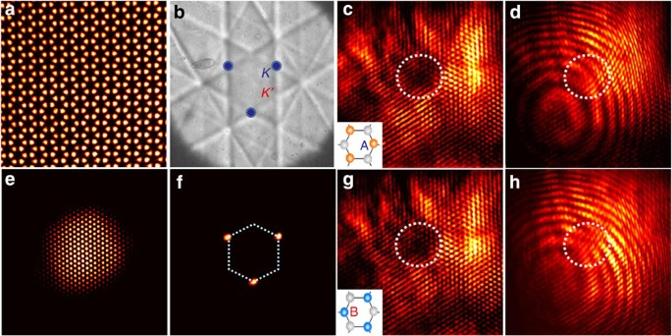Figure 3: Experimental observation of vortex generation by initial excitation of three Dirac points. (a) The honeycomb lattice optically induced in a nonlinear crystal, and (e) the probe beam at the input to the lattice containing no phase singularity. (b) Measured Brillouin zone spectrum of the induced lattice, and (f) thek-space spectrum of the input beam matching the three marked Dirac points inb. The white dashed lines mark the first BZ. (c,g) Output intensity patterns when only sublattice A (top row) or B (bottom row) is excited. The inserts illustrate the selective excitation of two sublattices by the probe beam corresponding toFig. 2, which leads to opposite vortex singularities as identified from the interferograms (d,h). Figure 3: Experimental observation of vortex generation by initial excitation of three Dirac points. ( a ) The honeycomb lattice optically induced in a nonlinear crystal, and ( e ) the probe beam at the input to the lattice containing no phase singularity. ( b ) Measured Brillouin zone spectrum of the induced lattice, and ( f ) the k -space spectrum of the input beam matching the three marked Dirac points in b . The white dashed lines mark the first BZ. ( c , g ) Output intensity patterns when only sublattice A (top row) or B (bottom row) is excited. The inserts illustrate the selective excitation of two sublattices by the probe beam corresponding to Fig. 2 , which leads to opposite vortex singularities as identified from the interferograms ( d , h ). 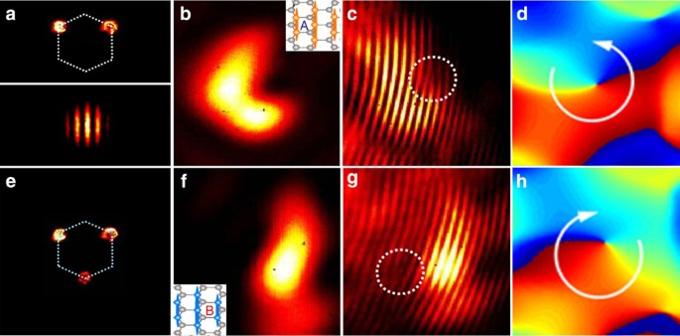Figure 4: Experimental observation of vortex generation by initial excitation of two Dirac points. (a) The input intensity pattern andk-space spectrum of the probe beam from two-beam interference, and (e) its output spectrum. Notice the new spectral component appearing at the third Dirac point due to Bragg reflection. (b,f) Output far-field intensity patterns generated at the third Dirac point when only sublattice A (top row) or B (bottom row) is excited. The insets illustrate the selective excitation of two sublattices by the probe beam. (c,g) Opposite vortex singularities observed from the interferograms ofbandf. (d,h) Output phase structure obtained from corresponding numerical simulation, where the opposite singularities are illustrated by the white arrows. Full size image Figure 4: Experimental observation of vortex generation by initial excitation of two Dirac points. ( a ) The input intensity pattern and k -space spectrum of the probe beam from two-beam interference, and ( e ) its output spectrum. Notice the new spectral component appearing at the third Dirac point due to Bragg reflection. ( b , f ) Output far-field intensity patterns generated at the third Dirac point when only sublattice A (top row) or B (bottom row) is excited. The insets illustrate the selective excitation of two sublattices by the probe beam. ( c , g ) Opposite vortex singularities observed from the interferograms of b and f . ( d , h ) Output phase structure obtained from corresponding numerical simulation, where the opposite singularities are illustrated by the white arrows. Full size image Pseudospin-mediated vortex generation by two-beam excitation In the second method, only two interfering beams are used as the probe, so only two Dirac points are initially excited ( Fig. 4a ). Nevertheless, due to the HCL symmetry and Bragg reflection, a new spectrum component emerges at the corresponding third Dirac point ( Fig. 4e ). Amazingly, the far-field intensity pattern of this new component (after a Fourier transform from momentum k -space back to real space) exhibits opposite vortex singularities as the two beams selectively excite sublattice A or B, revealed by the phase pattern obtained from both experimental interferogram ( Fig. 4c,g ) and numerical simulation ( Fig. 4d,h ). These results indicate again that the observed vortices and associated charge flipping arise from the honeycomb sublattice degree of freedom, that is, the pseudospin. Theoretical analysis with the Dirac equation To gain further insight of the underlying physics of pseudospin and unveil its AM, we directly analyse the normalized Dirac equation (equation (2)). Unlike the single-wavefunction description of the paraxial Schrödinger equation (equation (1)), the wave dynamics in the Dirac system is directly mapped into the two-component spinor wavefunction with components ψ A and ψ B . Consequently, there is absolutely no meaning in any form of interference between these two components. However, it is physically relevant to separate the wavefunction of the paraxial equation Ψ( r , z ) discretely according to its spatial location as and , where are the position vectors of the sublattice elements A and B with indices ( m , n ) located in the same Wigner-Seitz cell as . We introduce the total AM along z -direction as J = L + S , where is the orbital AM, S = μσ z /2 is the pseudospin ( μ =1 or −1, and σ z is the respective Pauli matrix), . The average total lattice AM with respect to the spinor wavefunctions ψ A and ψ B is then given by As an example, when μ =1, any excitation of sublattice A (or B) will have a positive (or negative) contribution to the total AM of the system. Typical numerical and analytical results obtained from the above Dirac equation are presented in Fig. 5a,b . Details of the calculations are given in the Supplementary Information section. To selectively excite a pseudospin eigenstate, we first separate the wavefunctions and the Floquet-Bloch modes discretely according to its spatial location in the two sublattices, and then solve the Dirac equation numerically with a Gaussian modulation of the separated Bloch modes as initial condition: , Ψ { B , A } ( r , z =0; μ )=0, where are the Floquet-Bloch modes localized at { A , B } lattice sites at K μ . Note that close to the six Dirac points m =1,…,6 the Floquet modes are degenerate when m =2 n , and m =2 n +1. Furthermore, even/odd values of m characterize opposite local phase structures such that . The respective optical field in the Dirac limit is then given by along with ψ { B , A } ( r , z )=0. At the input plane, the pseudospin is the only term that contributes to the total AM. However, from both the operator perspective (that is, expressing ( ∂ x + iμ∂ y ) in polar coordinates) and utilizing the Green’s function, it is clear that when the sublattice A (or B) is initially excited, the field in sublattice B (or A) will be generated with a topological charge μ (or − μ ). This is clearly illustrated in the numerical results of Fig. 5a . The asymptotic structure of the beam is derived by a combination of the steepest descent and stationary phase approximations (as detailed in the Supplementary Material ). 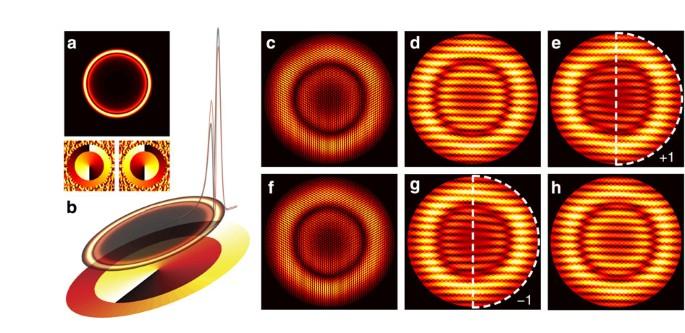Figure 5: Theoretical analysis of the pseudospin-mediated vortex generation. (a,b) Pseudospin-mediated vortex generation calculated directly from the Dirac equation. When only one of the spinor components ψA(ψB) is given an initial Gaussian-modulated excitation, the output intensity atz=30 is identical (top panel ofa) but the corresponding phase is different. The left (right) bottom panel ofashows the vortex phase ofψB(ψA), whereas the other component has uniform phase. Comparison between results from numerical solution (dark) and asymptotic calculation is shown inb. (c–h) Intensity and phase of the output optical field obtained from numerical simulation of the paraxial model with a graphene-type HCL potential based on decomposing the optical field into its spinor components. In the top (bottom) row, only sublattice A (B) is initially excited with a Gaussian modulation, which leads to similar intensity patterns (c,f) but opposite phase structures. The second column (d,g) shows the interferograms of the wavefunction ΨAand the third column (e,h) shows the corresponding interferograms of ΨB. These components ΨAand ΨBare derived by restricting the paraxial wavefuction Ψ to the discrete locations that are determined by the lattice elements A and B (see the relevant discussion in the text andSupplementary Informationsection). When the eigenstate of the lattice spin corresponding to A (B) is initially excited, a vortex is generated in the sublattice B (A) with a topological charge +1 (−1), respectively. For illustration purposes, we crop the area outside a disk that consists almost solely of the irrelevant plane-wave contribution. Specifically, when the sublattice A is initially excited, the analysis leads to Figure 5: Theoretical analysis of the pseudospin-mediated vortex generation. ( a , b ) Pseudospin-mediated vortex generation calculated directly from the Dirac equation. When only one of the spinor components ψ A (ψ B ) is given an initial Gaussian-modulated excitation, the output intensity at z =30 is identical (top panel of a ) but the corresponding phase is different. The left (right) bottom panel of a shows the vortex phase of ψ B ( ψ A ), whereas the other component has uniform phase. Comparison between results from numerical solution (dark) and asymptotic calculation is shown in b . ( c – h ) Intensity and phase of the output optical field obtained from numerical simulation of the paraxial model with a graphene-type HCL potential based on decomposing the optical field into its spinor components. In the top (bottom) row, only sublattice A (B) is initially excited with a Gaussian modulation, which leads to similar intensity patterns ( c , f ) but opposite phase structures. The second column ( d , g ) shows the interferograms of the wavefunction Ψ A and the third column ( e , h ) shows the corresponding interferograms of Ψ B . These components Ψ A and Ψ B are derived by restricting the paraxial wavefuction Ψ to the discrete locations that are determined by the lattice elements A and B (see the relevant discussion in the text and Supplementary Information section). When the eigenstate of the lattice spin corresponding to A (B) is initially excited, a vortex is generated in the sublattice B (A) with a topological charge +1 (−1), respectively. For illustration purposes, we crop the area outside a disk that consists almost solely of the irrelevant plane-wave contribution. Full size image which confirms the vortex generation in sublattice B. Likewise, when sublattice B is initially excited, due to the transformation ψ A ↔ ψ B , x →− x , y → y (holding for the Dirac system and thus for the above formulas), the optical field ψ A is generated with opposite vorticity − μ . As shown in Fig. 5b , the asymptotic calculations are in excellent agreement with numerical results. Importantly, both our calculation and simulation show that, at propagation distances where the conical diffraction becomes appreciable, the amplitude profiles of the two spinor components become identical, thus resulting in zero lattice spin as also seen from equation (3). In fact, the initial pseudospin is completely transferred to the final orbital AM of the system, that is, ‹ S › i = ‹ L › f . This explains the optical vortex (AM) generation in the HCL observed in our experiment. To substantiate our argument, we revisit the Schrödinger equation (equation (1)) with a HCL potential but perform numerical computations following the above procedure of decomposing the optical field into its spinor components. The results are shown in Fig. 5c–h , where the interferograms of the two components are examined separately. Evidently, when the spinor state A (or B) is excited, the initial positive (or negative) value of the total pseudospin is converted to a vortex AM with a topological charge +1 (or −1) carried completely by sublattice B (or A). Before closing, we emphasize that the total AM of the system J would not be conserved but should we ignore the pseudospin, simply because the orbital AM itself in the HCL is not conserved. In fact, the pseudospin represents the hidden AM due to the sublattice degree of freedom in the Dirac system of the HCL. The transverse derivatives associated with the Dirac equation (equation (2)) can be written as ∂ x ± i ∂ y = e ± iθ ( ∂ r −( i / r ) ∂ θ ), thus if one spinor component does not carry vorticity, the second spinor component is going to be ‘compatible’ only if its topological charge is +1 or −1. We note that our vortex generation and topological charge flipping is achieved by exciting the two sublattices at the same K valley (see Fig. 3 ) in a uniform (non-strained) HCL, thus no pseudomagnetic field is involved [22] . The observed pseudospin AM does not result from the valley-dependent nonzero Berry curvature at the K and K ′ valleys [34] . Experimentally, by exciting the same sublattice but from the two different sets of the valleys, we were unable to see any difference. Finally, we also mention that the concept of pseudospin could be extended to other types of lattices, such as the Kagome and Lieb lattices. In fact, with the Lieb lattices, it was recently suggested that the pseudospin is not merely a mathematical formality but rather has a physical effect [35] . In summary, we have demonstrated both theoretically and experimentally the pseudospin-mediated vortex generation in photonic graphene. Our results indicate clearly that the pseudospin is of real AM, observable and measurable. As this AM arises as a direct outcome of the Dirac equation also widely studied in graphene systems and topological insulators, we envisage our results will have broader impact to other branches of physics and material sciences. In addition, our work also brings about a new mechanism to generate optical vortices which may find applications in photonics. Optical induction and probing the photonic graphene The experimental setup (see Supplementary Fig. 1 ) relies on the optical induction method [14] , [29] , [30] , which leads to a honeycomb pattern of refractive index change in a nonlinear photorefractive crystal. We probe the pseudospin states by launching three or two interfering beams as the probe to the HCL, and monitor the output transverse intensity pattern and the phase of the probe exiting the lattice. To do so, we use a beam from an argon-ion laser operating at 488 nm wavelength and split it into two beams, one being ordinarily polarized for ‘writing’ the HCL pattern into the crystal and the other being extra-ordinarily polarized for probing the pseudospin states. The writing beam passes through a rotating diffuser, turning into partially spatial incoherent, before it is sent through a specially designed amplitude mask. The mask generates either three interfering beams that together generate a triangular lattice interference pattern, or six interfering beams that generate a HCL pattern. Such intensity patterns remain invariant during propagation through the crystal. For the experiment of Fig. 3 , the HCL was generated by employing the self-defocusing nonlinearity on the triangular intensity pattern [14] , as used in our previous work with graphene edge states [20] . In this case, the refractive index pattern is the ‘negative’ of the intensity pattern of the lattice-inducing beam. For the experiment of Fig. 4 , the HCL was generated by employing the self-focusing nonlinearity on the honeycomb intensity pattern, so in this latter case, the refractive index pattern matches the intensity pattern directly [36] . In both cases, a honeycomb pattern of waveguide arrays (photonic graphene) is established, with the same structure as shown in the left insert in Supplementary Fig. 1 . The probe beams, either by interfering three beams to a triangular pattern as for Fig. 3 or by interfering two beams to a linear fringe-like pattern as for Fig. 4 , are affected by the induced HCL and propagate under the influence thereof. In our experiment, the probe beams are appropriately focused and fine-tuned so they are aimed into the desired Dirac points in the first Brillouin zone of the HCL as shown in the right insert in Supplementary Fig. 1 . How to cite this article: Song, D. et al. Unveiling pseudospin and angular momentum in photonic graphene. Nat. Commun. 6:6272 doi: 10.1038/ncomms7272 (2015).